Molecular adsorption induces the transformation of rhombohedral- to Bernal-stacking order in trilayer graphene The Bernal (ABA)-stacked graphene trilayer is presumed to be thermodynamically more stable than the rhombohedral (ABC) counterpart. However, the thermal transformation from ABC to ABA domains does not occur at a temperature lower than 1,000 °C. Here we report that ABC-stacked trilayers are transformed to ABA-stacked layers after an organic molecule triazine is evaporated onto graphene surfaces at 150 °C. The transformation is found to always initiate at the ABA–ABC domain boundaries. Simulations based on density function theory considering the van der Waals interaction suggest that after triazine decoration the energy difference between ABA and ABC domains is larger, providing a driving force for stacking transformation. The molecular dynamics simulation results further suggest that the triazine decoration on the wrinkles at the ABC–ABA domain boundary activates the wrinkle sliding toward the ABC domains, leading to the stacking transformation from ABC to ABA. Single-layer and bilayer graphene sheets have stimulated intense interest because of their unique electronic structures [1] , [2] , [3] , [4] and great potential for various applications, such as high-frequency devices, [5] flexible electronics [6] , [7] and sensors [8] , [9] . Few-layer graphene sheets, including trilayer and other thicker graphene layers, have recently attracted increasing attention [10] , [11] , [12] , [13] , [14] , [15] , [16] , because the crystallographic stacking order of individual graphene sheets provides an additional parameter for tuning their electronic properties [17] , [18] , [19] , [20] , [21] . The rhombohedral (ABC) and Bernal (ABA) stacking orders are two stable crystallographic configurations. These graphene trilayers are expected to exhibit different phenomena at low charge densities because of various layer-to-layer electronic interactions and competing symmetries [15] . The ABA-stacking order is slightly more thermodynamically stable than the ABC-stacking order. However, the ABC graphite was found to retain its stacking order, even at a temperature as high as 1,000–1,200 °C (refs 22 , 23 ). These results indicate a significant energy barrier for configuration transformation from the ABC to ABA-stacking order. Lui et al. [17] demonstrated that the Raman 2D peak shape of the ABC-stacked graphene trilayer (and tetralayer) was distinctively different from that of the ABA-stacked layer, where the full-width at half maximum (FWHM) of the ABC-stacked few-layer graphene was ~10 cm −1 broader as compared with the ABA-stacked graphene. Cong et al. [24] reported that the M band at ~1,740 cm −1 is a single and asymmetric peak in the ABA-stacked trilayer, but it splits into two peaks in the ABC-stacked trilayer. These studies provide a simple and useful methodology for characterizing the ABC- and ABA-stacked domains by Raman spectroscopy. In this contribution, a layer of small organic molecules 1,3,5-triazine (abbreviated as triazine) was deposited onto mechanically exfoliated few-layer graphene by vapour evaporation at only 150 °C. After triazine decoration, certain ABC-stacked domains were transformed to ABA-stacked domains. This was confirmed by the changes in three Raman vibration modes of 2D, M and G bands. The experiments revealed that the transformation always started at the ABA–ABC domain boundaries, where the domain conversion (growth of ABA from ABC domains) is analogous to the conventional crystal growth process. 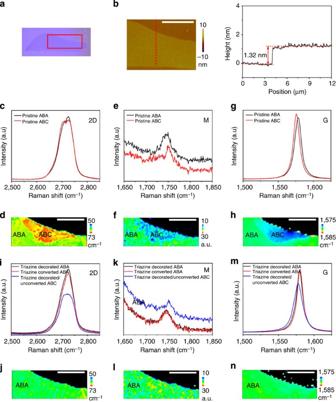Figure 1: Characterization of ABC and ABA domains using Raman spectroscopy. (a) The optical micrograph of a graphene trilayer with ABA and ABC domains. (b) The AFM height image for the around ABC-stacked area of the red square in (a). The cross-sectional height along the dotted line in (b) shows on the figure to the right that there is no height difference between ABA and ABC domains. (c,e,g) Raman 2D, M and G-band spectra, respectively, for the pristine ABA- and ABC-stacking domains. (d,f,h) Raman mappings of the pristine trilayer constructed using FWHM of 2D band, integrated M-band peak area and G-band frequency, respectively. (i,k,m) Raman 2D, M and G-band spectra, respectively, for the triazine decorated ABA, triazine converted ABA and triazine decorated/unconverted ABC-stacking domains. (j,l,n) Raman mappings of the sample after triazine decoration, constructed using 2D FWHM, integrated M-band peak area and G-band frequency, respectively. The scale bar length on the right of the AFM and mappings, 10 μm. Identification of ABC and ABA domains Figure 1a shows the optical micrograph for a graphene flake obtained by micromechanical exfoliation. Figure 1b presents the atomic force microscopy (AFM) topology for the graphene flake, indicated as the selected squared area in Fig. 1a . The AFM image in Fig. 1b shows that the selected sample is a trilayer graphene with uniform thickness (1.32 nm) across the whole area. The Raman 2D mode, arising from an inter-valley double-resonant process that involves two in-plane transverse optical phonons near the K point in the Brillouin zone, is sensitive to the electronic structure of graphene [23] . Its line shape provides an accurate signature of the AB-stacked bilayer graphene [25] , [26] . Lui et al. [17] demonstrated that the 2D bandwidth of the ABC-stacked few-layer graphene was broader than that of the ABA-stacked graphene. Figure 1c displays the Raman 2D peak profiles, excited by a 473-nm laser, for the graphene flake shown in Fig. 1b . The flake also consists of two types of Raman 2D shapes, which corresponds to ABA- and ABC-stacked graphene trilayers. The 2D FWHM of the ABA-stacking order is ~8 cm −1 smaller than that of the ABC-stacking order. Lui et al. [17] suggested fitting the 2D spectrum at each pixel of the spatial mapping to a single Lorenzian function. Displaying the FWHM of the fitted Lorenzian peak for each pixel visualizes the spatial distribution of the ABC- and ABA-stacked domains. Figure 1d shows the Raman 2D FWHM mapping of the trilayer flake based on Lui’s method. Two distinct areas are identified as the ABA- and ABC-stacked domains. These two areas are undistinguishable in the AFM height image ( Fig. 1b ). In addition to the 2D FWHM, the Raman M band at ~1,740 cm −1 , which has been assigned to the second-order overtone of the out-of-plane transverse mode [25] , [26] , is also the fingerprint of the interlayer coupling effect. The M band is activated by the strong coupling between the graphene layers, and thus, it is observed in the AB-stacked graphene bilayer and absent in both the monolayer graphene and the incommensurate bilayer graphene [23] , [25] , [26] . Cong et al. [24] have recently shown that the M band at ~1,740 cm −1 exhibits a single peak in the ABA-stacked trilayer, but it splits into two peaks in the ABC-stacked trilayer. Figure 1e shows the Raman M-band features for the identified ABA- and ABC-stacked trilayers obtained from the same flake. The M band for the ABA domain has a single peak and is centred at 1,746 cm −1 , whereas it splits into two peaks (1,735 and 1,751 cm −1 ) in the ABC domain, consistent with the experimental observation by Cong et al. [24] Supplementary Figure S1 provides the M-band characteristics for the bilayer, trilayer and tetralayer graphene. The integrated peak area of the split M bands from the ABC-stacked domain is smaller than that of the ABA-stacked domain, and the false colour spatial mapping constructed by plotting the M peak area also allows visualizing the spatial distribution of ABA- and ABC-stacked domains, as shown in Fig. 1f . Figure 1g shows that the G peak frequency for the ABA-stacking order is 3 cm −1 higher than that of the ABC-stacking order, consistent with the report by Lui et al. [17] . The ABC- and ABA-domain distribution identified by the integrated M peak area or G-band frequency is the same as that identified by the 2D FWHM. Figure 1: Characterization of ABC and ABA domains using Raman spectroscopy. ( a ) The optical micrograph of a graphene trilayer with ABA and ABC domains. ( b ) The AFM height image for the around ABC-stacked area of the red square in ( a ). The cross-sectional height along the dotted line in ( b ) shows on the figure to the right that there is no height difference between ABA and ABC domains. ( c , e , g ) Raman 2D, M and G-band spectra, respectively, for the pristine ABA- and ABC-stacking domains. ( d , f , h ) Raman mappings of the pristine trilayer constructed using FWHM of 2D band, integrated M-band peak area and G-band frequency, respectively. ( i , k , m ) Raman 2D, M and G-band spectra, respectively, for the triazine decorated ABA, triazine converted ABA and triazine decorated/unconverted ABC-stacking domains. ( j , l , n ) Raman mappings of the sample after triazine decoration, constructed using 2D FWHM, integrated M-band peak area and G-band frequency, respectively. The scale bar length on the right of the AFM and mappings, 10 μm. Full size image Domain transformation The ABA-stacking order is slightly more thermodynamically stable compared with the ABC-stacking order [27] , [28] . The lateral energy barrier between these two stackings has been calculated to be ~2 meV per atom [29] . A recent study confirmed that the ABC-stacked graphene trilayer was stable after annealing at 800 °C (ref. 19 ). Previously, we have found that an organic molecule, triazine can be adsorbed and form a uniform layer on bilayer graphene, resulting in the band-gap opening by breaking the inversion symmetry between the top and bottom layers [30] . With this inspiration, we thermally evaporated triazine molecules on the ABC-stacked graphene trilayer at 150° for 8 h. Figure 1i shows the Raman 2D spectra of the ABA- and ABC-domains for the same flake after triazine decoration, where the FWHM of the previously identified ABC domain is obviously narrowed, and the peak shape becomes undistinguishable to the ABA domains. The Raman spectrum for the unconverted ABC domains after triazine decoration was also included for comparison from another trilayer flake on the same substrate. The unconverted ABC domain still exhibits a broader FWHM after triazine decoration. Figure 1k demonstrates that the double-peaked M band in pristine ABC domains has been changed to a single peak after triazine decoration. Similarly, the G-band frequency for the ABC domain has become the same as that for the ABA domain after triazine decoration, as shown in Fig. 1m . The Raman mappings for 2D FWHM, the integrated M-band area and the G-band frequency shown in Fig. 1j clearly shows that the ABC-stacking domain has been changed to an ABA domain, where the false colour scale for each mapping is the same as in the corresponding Fig. 1d . This study performed the 150 °C triazine decoration experiments for seven samples, and the transformation was observed in all samples. The transformation probability is 41.3% on average. A higher decoration temperature of 250 °C results in a lower (9.6%) transformation, because the desorption of triazine molecules from the graphene surface is faster at higher temperatures (see Supplementary Table S1 for details). We have tested two other commonly used molecules, tetracyanoquinodimethane and melamine, known to exhibit strong interaction with graphene. However, no stacking transformation was observed. The results in Fig. 1 suggest that the Raman mapping of the 2D FWHM suffices in efficiency to differentiate between the ABA and ABC domains. As the intensity of the 2D band is strong, 2D FWHM Raman mapping was used to further reveal the details of the stacking order transformation. 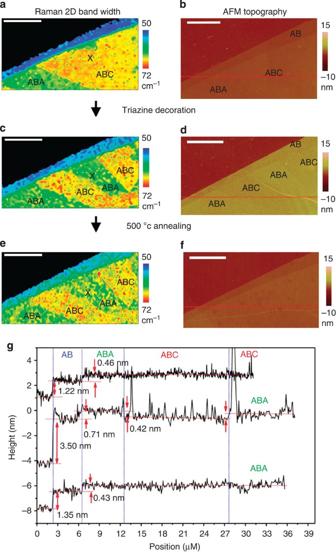Figure 2: Transformation of stacking order in trilayer graphene. (a,c,e) Raman mappings of the FWHM of 2D band before and after triazine decoration, and after triazine removal by 500 °C annealing, respectively. The black dotted line is to guild to visualize the boundaries between the ABA and ABC domains.b,d,fAre the AFM images corresponding to the Raman mapping areas in thea,c,e, respectively. (g) The AFM height profiles for a selected line across the ABA and ABC domains. The scale bars on the left of (a–f), 10 μm in length. Figure 2a shows the Raman 2D FWHM map and the AFM topology image for the selected area of another graphene flake before triazine deposition. Figure 2c shows the corresponding Raman map and AFM image after triazine decoration. The ABA domains remain as ABA after triazine deposition. However, the location labelled with a ‘cross’ sign originally identified as the ABC-stacking order has been transformed to ABA-stacking, directly proving that the ABA-stacking order is thermodynamically more stable than the ABC-stacking order. The newly formed ABA domain starts from the small ABA domain (the green triangle area in Fig. 2a ). Supplementary Figure S2 provides another example showing that the conversion started from ABA domains. To ensure that the 2D and M-band changes after triazine deposition are not the artifact caused by triazine, the triazine layer was removed by annealing at 500 °C (in Ar for 5 h). Supplementary Figure S3a,b shows the 2D and M bands for the converted domain before and after triazine removal, respectively. The line shape of the 2D band and the M-band profile remain unchanged, corroborating that the ABC-stacked domain was transformed to an ABA-stacked domain. Figure 2e shows the corresponding Raman map and AFM image after triazine removal, where the AFM topography of the whole area becomes flat again because of the removal of triazine molecules. However, the ABA and ABC domain distribution is the same as before triazine removal. Figure 2: Transformation of stacking order in trilayer graphene. ( a,c , e ) Raman mappings of the FWHM of 2D band before and after triazine decoration, and after triazine removal by 500 °C annealing, respectively. The black dotted line is to guild to visualize the boundaries between the ABA and ABC domains. b , d , f Are the AFM images corresponding to the Raman mapping areas in the a , c , e , respectively. ( g ) The AFM height profiles for a selected line across the ABA and ABC domains. The scale bars on the left of ( a – f ), 10 μm in length. Full size image Morphology of ABA and ABC domains Figure 2g shows the height profiles of a selected line across the ABA- and ABC-stacked areas shown in Fig. 2b . The top trace shows that the ABA- and ABC-stacked domains are of similar height and undistinguishable in the AFM topological image. After triazine decoration, the thickness of the AB bilayer area increases from 1.22 to 3.5 nm, and the height difference between the AB bilayer and the ABA trilayer increases from 0.46 to 0.71 nm. After triazine decoration, the ABA-stacked trilayer domain is 0.42 nm thicker than the ABC-stacked trilayer domain. These results corroborate that a triazine layer was deposited onto the graphene surfaces. The AFM topological image of the ABA- and ABC-stacked domains ( Fig. 2d ) corresponds well to the mapping of the Raman 2D bandwidth ( Fig. 2c ), meaning that the AFM topological image after triazine decoration could also be used to visualize the spatial distribution of ABA- and ABC-stacked domains. We have compared the total energies of a triazine molecule adsorbed parallel to or perpendicularly on a trilayer graphene sheet for both ABA and ABC-stacking forms, as shown in Supplementary Table S2 . Our results show that a triazine molecule prefers to absorb parallel to a trilayer graphene sheet. To further clarify the effect of triazine decoration, this study performed density functional theory (DFT) simulations to examine whether the ABC to ABA domain transformation is energetically favourable. As shown in Supplementary Table S3 , the local-density approximation calculations show that the energy difference between pristine ABA and ABC-stacking domains is 4 meV, which increases to 8 meV after triazine decoration. When considering the van der Waals (vdW) correction by using the vdW density function, the energy difference is 35 meV before decoration and 68 meV after decoration. As a benchmark, the difference in total energies was compared between the ABA-stacking and the ABC-stacking graphite by employing the adiabatic-connection fluctuation-dissipation theorem within random-phase approximation (ACFDT-RPA). The RPA results show that the total energy of the ABA-stacking form is 1 meV per unit cell lower than that of the ABC-stacking form, consistent with standard DFT methods. Meanwhile, triazine molecules always adopt the C-top configuration, where the N atoms stay above the hollow of carbon rings in the top graphene layer. For the ABA domain, it means that the triazine molecules form a new fourth layer with ABA-like stacking (that is, ABAB). For the ABC domain, the fourth triazine layer combined with the underlying ABC trilayer graphene forms ABCA or ABCB configurations, which may be an intuitive explanation for the increased energy difference. These results suggest that the enlarged energy difference between ABA and ABC domains after triazine decoration provides a driving force for the transformation of ABC to ABA domains at low temperatures. To explore the physical mechanism responsible for the observed ABC- to ABA-domain transformation, this study conducted a simulation by using the density functional tight binding-molecular dynamics method. The possible stacking sequences in the ABA/ABC sample are critical for the simulation and discussion. 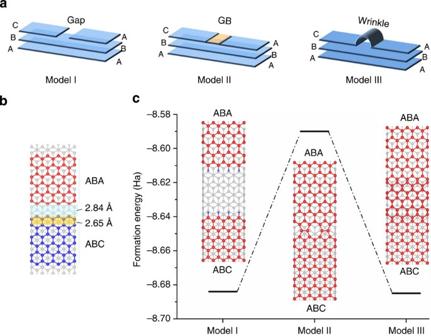Figure 3: Proposed models for constructing graphene trilayers. (a) Schematic illustration for three possible ways of constructing an ABA/ABC graphene trilayer. Model I: ABA/ABC separated by a gap. Model II: ABA/ABC separated by GB defects. Model III: ABA/ABC separated by a wrinkle. (b) To construct a ABA/ABC domain structure, the carbon atoms between ABA and ABC domains must shift by 2.84+2.65 ×nÅ (n=0, 1, 2, 3,...) along the armchair direction. (c) The formation energies (Ef) for all these three possible configurations, Model I, II and III.Ef=Esystem−mEC−nEH, whereECandEHdenote the energies of bulk graphite and hydrogen molecule. Figure 3a schematically shows the three possible ways of constructing an ABA/ABC sample. In the following discussion, to construct an ABA/ABC domain structure, the carbon atoms between ABA and ABC domains must shift by 2.84+2.65 × n Å ( n =0, 1, 2, 3,...) along the armchair direction, as shown in Fig. 3b , where 2.84 Å equals two times the C–C bond length. Model I represents a gapped ABA/ABC trilayer, which consists of a continuous ABA-stacked AB bilayer with the additional A layer and C layer on top separated by a small gap. Model II is the grain boundary (GB) separated by the ABA/ABC trilayer, which consists of the ABA and ABC domains separated by a GB. GBs primarily consist of pentagon and heptagon pairs, and occasionally octagon rings to reconcile the connection of the two domains. Model III is the wrinkle-separated ABA/ABC trilayer, where the ABA and ABC domains are constructed from a continuous graphene layer. In this model, it is necessary to have a wrinkle separating the two domains to accommodate the 2.84+2.65 × n Å shift between the two stacking orders. Both Raman and AFM do not have a sufficiently high spatial resolution to differentiate between these models. However, simulations can help in understanding the transformation processes. We calculated the formation energies for the three possible configurations that contain both ABA and ABC domains, as shown in Fig. 3c . Formation energy is defined as E f = E system − mE C − nE H , where E C and E H denote the energies of bulk graphite and the hydrogen molecule, respectively. As expected, the domains separated by point defects (Model I), such as the 5-5-8-5-5 GB, are energetically unfavourable compared with other models. This study adopted n =0 in calculating formation energy because the other case (that is, n >0) contains more defects and is less stable. Point defects (for example, vacancies and interstitials) can be trapped by the strained GB region, which in turn facilitates the migration of a GB in numerous samples, but has not been reported for graphene samples. Cong et al. [24] reported that in one of their graphene trilayer samples, they observed tensile strain that induced G and 2D phonon softening at the ABC and ABA domain boundary [31] , [32] , [33] , [34] . However, the migration of GB in graphene is difficult because it requires the constant breaking and reforming of the C layer in the pentagon and heptagon rings. The diffusion and coalescence of vacancies in the GB region require a temperature of 2,000 K, which is substantially higher than the temperature used in this study [35] . Hence, this model is highly unlikely, and can be excluded. For the wrinkle-separated ABA/ABC trilayer (Model III), a wrinkle was first made for the top-layer graphene, and the energy of the trilayer was minimized using a DFT calculation, showing that the separation using n =3 is the most stable structure. The gapped ABA/ABC trilayer (Model I) is also made with n =3 for a fair comparison with Model I. The results show that Model III exhibits a similar formation energy compared with Model I. Figure 3: Proposed models for constructing graphene trilayers. ( a ) Schematic illustration for three possible ways of constructing an ABA/ABC graphene trilayer. Model I: ABA/ABC separated by a gap. Model II: ABA/ABC separated by GB defects. Model III: ABA/ABC separated by a wrinkle. ( b ) To construct a ABA/ABC domain structure, the carbon atoms between ABA and ABC domains must shift by 2.84+2.65 × n Å ( n =0, 1, 2, 3,...) along the armchair direction. ( c ) The formation energies ( E f ) for all these three possible configurations, Model I, II and III. E f = E system − mE C − nE H , where E C and E H denote the energies of bulk graphite and hydrogen molecule. Full size image The MD simulation in Fig. 4a shows that, when considering the triazine adsorption on the wrinkle-separated ABA/ABC trilayer, the triazine molecules on top of the wrinkle region show tilting, which acts as a driving force to the wrinkle, leading the wrinkle to move toward the ABC domain direction, causing instability of the ABC domain. As shown in Fig. 4b , for the ABA domain, the atomic arrangements do not show a significant change. Compared with the stable ABA domain, the atomic lattice of the C layer in the ABC domain presents obvious slipping. The atoms in the top layer of the ABC domain shift from their original position, induced by the slight movement of the wrinkle, resulting in the final transformation of the ABC to ABA domains. However, for Model I, to explain the crystal growth-like behaviour for the ABC to ABA transformation observed in Fig. 2 , the shift of the carbon atoms of the top-layer graphene from the edge of the ABC domain should result in an increased gap area, which is apparently not observed in our experiment. Thus, Model I is excluded. Combined with the experimental observation of a gradual ABC to ABA transformation, the structure with a wrinkle separating the ABA and ABC domains is the most plausible stacking sequence. 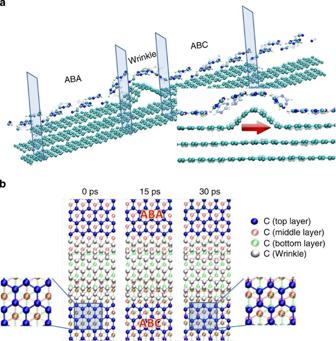Figure 4: Molecular dynamics simulations. The structural transformation of trilayer graphene decorated with triazine molecules at 500 K. (a) Structural evolution of the system between the initial model at 0 ps, (solid trace) and the structure at 30 ps (shaded trace). The simulated system contains an ABA domain and an ABC domain with a wrinkle, decorated with a single layer of triazine molecules. Inset: magnified plot around the wrinkle. The red arrow indicates that the wrinkle moves towards the ABC domain direction, causing the instability of the ABC domain. During the process, the triazine molecules on the top of the wrinkle show tilting, which act as a driving force to the wrinkle, leading to the wrinkle movement predominately towards the side of the ABC domain. Atomic colours are as follows: H, white; N, blue; C, cyan. (b) Top-view snapshots of trilayer graphene (Top layer: blue; Middle layer: red; Bottom layer: green) near the wrinkle (white region). For clarity, the triazine molecules are not shown. The insets show the atomic configurations of the ABC domain at 0 and 30 ps. At 0 ps, the atoms in the bottom layer are all completely masked by those in the middle and top layers, while at 30 ps, the atoms in the top layer shift from their original position induced by the orientational change of the triazine molecules. For the ABA domain, the atomic arrangements do not show significant change. Figure 4: Molecular dynamics simulations. The structural transformation of trilayer graphene decorated with triazine molecules at 500 K. ( a ) Structural evolution of the system between the initial model at 0 ps, (solid trace) and the structure at 30 ps (shaded trace). The simulated system contains an ABA domain and an ABC domain with a wrinkle, decorated with a single layer of triazine molecules. Inset: magnified plot around the wrinkle. The red arrow indicates that the wrinkle moves towards the ABC domain direction, causing the instability of the ABC domain. During the process, the triazine molecules on the top of the wrinkle show tilting, which act as a driving force to the wrinkle, leading to the wrinkle movement predominately towards the side of the ABC domain. Atomic colours are as follows: H, white; N, blue; C, cyan. ( b ) Top-view snapshots of trilayer graphene (Top layer: blue; Middle layer: red; Bottom layer: green) near the wrinkle (white region). For clarity, the triazine molecules are not shown. The insets show the atomic configurations of the ABC domain at 0 and 30 ps. At 0 ps, the atoms in the bottom layer are all completely masked by those in the middle and top layers, while at 30 ps, the atoms in the top layer shift from their original position induced by the orientational change of the triazine molecules. For the ABA domain, the atomic arrangements do not show significant change. Full size image In summary, this work explores that the deposition of triazine molecules on top of the graphene trilayers results in the transformation of certain ABC-stacked to ABA-stacked domains, which was confirmed by changes in the Raman 2D, M and G bands. This observation directly proves that the ABA-stacked graphene trilayer is thermodynamically more stable than the ABC-stacked counterpart. The transformation of ABC to ABA domains started at the ABA–ABC domain boundaries. The calculations show that after triazine decoration, the energy difference between the ABA and ABC domains is larger, providing a driving force for stacking transformation. The structure with a wrinkle separating the ABA and ABC domains is the most plausible ABA–ABC domain boundary structure for the samples, and the triazine molecular decoration on the wrinkled graphene at the ABC–ABA domain boundary activates the wrinkle movement toward the ABC domains, resulting in ABA domain growth and a stacking transformation of ABC to ABA. The triazine-induced ABC- to ABA-stacking transformation was also observed for thicker graphene layers such as tetra-layers and hexa-layers (see Supplementary Fig. S4 for details). Although the details of the transformation from ABC- to the ABA-stacking order for thicker graphene layers remain under investigation, the activation of top-layer wrinkles by triazine molecule decoration may also affect the structural property of graphene layers underneath, which could result in the rearrangement of the stacking order in few-layer graphene. Sample preparation Graphenes were mechanically exfoliated from natural graphite flakes (purchased from NGS) and then transferred to a substrate with 300 nm SiO 2 on highly doped Si. We verified the graphene layers using optical microscopy, Raman spectroscopy and AFM. From Raman 2D profiles, we did not observe turbostatic structure in our exfoliated trilayer samples. After characterization, the 1,3,5-triazine was thermally evaporated onto graphene films at 150 °C. The evaporation period was around 8 h. The setup and process are the same to the reference [30] . Characterization The AFM images were performed in a Veeco Dimension-Icon system. Raman spectra were collected in a confocal Raman system (NT-MDT). The wavelength of laser is 473 nm (2.63 eV), and the spot size of the laser beam is ~0.5 μm. The step size of Raman spatial mapping is 0.5 μm, and the spectral resolution is 3 cm −1 (obtained with a 600-grooves per mm grating). A high grating (1,800 grooves per mm) is also used to get more details of line shapes of Raman band, and the spectral resolution is 1 cm −1 . The Si peak at 520 cm −1 was used as a reference for wavenumber calibration. Simulation For the simulation study, trilayer graphene flakes with a wrinkle GB were calculated by the density functional tight binding-molecular dynamics method [36] , [37] . The simulation system is coupled to an Andersen thermostat in order to maintain an invariant temperature of 500 K. A small time step of 0.1 fs is adopted to ensure the integration stability for the higher frequency C–H stretch vibrations. The model containing 1,076 atoms was initially constructed according to the reliability. The triazine molecules are adopted with the most stable configurations for ABC and ABA domains, where carbon atoms in triazine molecules overlap with the graphene lattice. The vdW interaction between the atoms is taken into account via a Lennard–Jones potential. The first-principles DFT calculations to compute the total energies of systems are performed with the plane wave basis Vienna ab initio simulation pack (VASP) code [38] . The electron–ion interaction was described using a projector augmented wave method and the exchange correlation potential was described using the local-density approximation in the parametrization of Perdew and Zunger [39] . We accounted for the non-local correlation energies by employing the vdW density functional method [40] . A kinetic energy cutoff at 400 eV was adopted. As a benchmark, we calculated the energy difference between the ABA stacking and ABC-stacking graphite employing the ACFDT-RPA using VASP [41] , [42] , [43] . Here, the in-plane lattice parameter and the interplane distance along the stacking direction is set to the experimental value of 2.46 and 3.34 Å. To ensure the convergence, we used high plane wave cutoffs of 800 eV both for the Hartree–Fock part and the correlation part [44] , [45] . For the HF part, 26 × 26 × 8 k-grid was used. Results are shown in Supplementary Fig. S5 . How to cite this article: Zhang, W. et al. Molecular adsorption induces the transformation of rhombohedral- to Bernal-stacking order in trilayer graphene. Nat. Commun. 4:2074 doi: 10.1038/ncomms3074 (2013).